Promotion of behavior and neuronal function by reactive oxygen species inC.elegans Reactive oxygen species (ROS) are well known to elicit a plethora of detrimental effects on cellular functions by causing damages to proteins, lipids and nucleic acids. Neurons are particularly vulnerable to ROS, and nearly all forms of neurodegenerative diseases are associated with oxidative stress. Here, we report the surprising finding that exposing C. elegans to low doses of H 2 O 2 promotes, rather than compromises, sensory behavior and the function of sensory neurons such as ASH. This beneficial effect of H 2 O 2 is mediated by an evolutionarily conserved peroxiredoxin-p38/MAPK signaling cascade. We further show that p38/MAPK signals to AKT and the TRPV channel OSM-9, a sensory channel in ASH neurons. AKT phosphorylates OSM-9, and such phosphorylation is required for H 2 O 2 -induced potentiation of sensory behavior and ASH neuron function. Our results uncover a beneficial effect of ROS on neurons, revealing unexpected complexity of the action of oxidative stressors in the nervous system. Reactive oxygen species (ROS) cause a wide range of detrimental effects at the cellular level, leading to protein aggregation, aberrant cell signaling, and ultimately cell senescence and death [1] , [2] . They do so by oxidizing cellular components such as proteins, lipids and nucleic acids, as well as via cellular signaling [1] , [3] . Exposure to ROS also triggers defense mechanisms in the cell by up-regulating the production of antioxidants that remove ROS (ref. 2 ). An imbalance between ROS production and removal results in oxidative stress [2] . Neurons are among the cell types that are most vulnerable to oxidative insults, largely due to their high metabolic rate and low regenerative potential [2] , [4] . The deleterious role of ROS in the nervous system has been well documented. For example, the progression of neurodegenerative diseases, such as Alzheimer’s disease, Parkinson’s disease and amyotrophic lateral sclerosis, is associated with oxidative stress [2] , [4] . Ischemia, seizure, and traumatic brain injury all trigger excess production of ROS, which contribute to the brain damages caused by these pathophysiological conditions [2] , [4] . Notwithstanding the detrimental impact of ROS, these agents are produced in cells under physiological conditions, such as mitochondrial respiration and innate immune response, and regulate cellular signaling [3] , [5] . For example, an increase in the production of ROS by mitochondria may induce adaptive responses and subsequently potentiate stress resistance in animals, a phenomenon called mitohormesis [6] , [7] . This led us to question if ROS have other types of effects on brain function. Here, we explore this possibility in the nematode Caenorhabditis elegans , a popular genetic model organism with a nervous system that has been very well characterized. We find that while high concentrations of H 2 O 2 are detrimental to C. elegans , low doses of H 2 O 2 , surprisingly, promote sensory behavior and also potentiate sensory neuronal function. Reducing the level of endogenous H 2 O 2 produces an opposite effect, suggesting that the effect of H 2 O 2 is physiological. The beneficial role of H 2 O 2 is mediated by an evolutionarily-conserved peroxiredoxin-p38/MAPK signaling axis that signals to AKT and the sensory channel TRPV/OSM-9. We further show that AKT regulates TRPV/OSM-9 sensory channel through phosphorylation. These findings reveal a beneficial effect of ROS on nervous system function. Low doses of H 2 O 2 promote sensory behavior Despite its small size, C. elegans nervous system drives a rich repertoire of behaviors, particularly sensory behaviors [8] . Previous work examining the role of ROS on worm behavior has mainly focused on high doses of H 2 O 2 , and found that exposing worms to the millimolar range of H 2 O 2 severely compromises behavior [9] . We thus started by testing a wider range of concentrations of H 2 O 2 ( Fig. 1a ). We incubated worms with varying concentrations of H 2 O 2 , and after a brief recovery, we examined their behavioral responses to sensory cues (see Materials and Methods). We focused on osmotic avoidance behavior, one of the best characterized sensory behaviors in C. elegans (ref. 8 ). Treating worms with 1 mM H 2 O 2 suppressed osmotic avoidance behavior by decreasing their response rate to high osmolarity solution (glycerol) ( Fig. 1a and Supplementary Fig. 1 ), consistent with the notion that oxidative insults negatively affect worm behavior [9] . Surprisingly, exposing worms to lower concentrations of H 2 O 2 at the micromolar and sub-micromolar range potentiated osmotic avoidance behavior ( Fig. 1a and Supplementary Fig. 1 ). Treatment with H 2 O 2 for 1 h was sufficient to induce such behavioral potentiation ( Fig. 1b ). Exposing worms to the ROS-producing agent paraquat also elicited similar effects ( Supplementary Fig. 2a ), while heat treatment did not ( Supplementary Fig. 2b ). Osmotic avoidance behavior is mediated by the polymodal sensory neuron ASH which detects high osmolarity cues [10] , [11] . This neuron also mediates octanol avoidance response [12] , and we obtained similar results with octanol avoidance behavior in worms treated with H 2 O 2 ( Supplementary Fig. 2c ). These experiments reveal a beneficial role of H 2 O 2 in promoting behavioral responses in C. elegans . 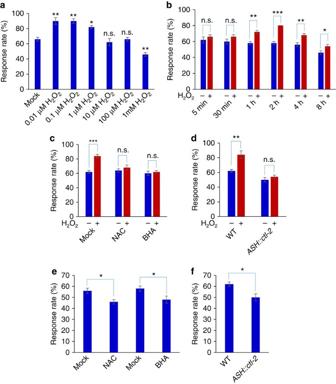Figure 1: Low doses of H2O2promote osmotic avoidance behavior. (a) Low doses of H2O2promote osmotic avoidance behavior while high concentrations of H2O2inhibit it. Worms were pre-incubated with varying concentrations of H2O2for 2 h. After a brief recovery on seeded NGM plates (up to 2 h), worms were tested for avoidance response to glycerol. To avoid a ceiling effect which would mask behavioral potentiation, a non-saturating concentration of glycerol (0.5 M) was used to challenge the worm.n≥20; *P<0.05, **P<0.005 (ANOVA with Dunnett’s test); Error bars: s.e.m. (b) Exposing worms to H2O2for one hour is sufficient to induce behavioral potentiation. Worms were pre-treated with 0.1 μM of H2O2for varying durations of time.n≥20; *P<0.05, **P<0.005, ***P<0.0005 (ttest); Error bars: s.e.m. (c) The antioxidants NAC and BHA block H2O2-induced behavioral potentiation. BHA (butylated hydroxyanisole, 25 μM) and NAC (N-acetyl-cysteine, 1 mM) were included during H2O2(0.1 μM ) treatment.n≥10; ***P<0.0005 (ANOVA); Error bars: s.e.m. (d) Transgenic expression of the catalase genectl-2in ASH neurons blocks H2O2-induced behavioral potentiation. H2O2: 0.1 μM. Thesra-6promoter was used to drive expression ofctl-2in ASH neurons.n≥10; **P<0.005 (ANOVA); Error bars: s.e.m. (e) Reducing the level of endogenous H2O2suppresses osmotic avoidance behavior. Worms were treated with BHA or NAC for 2 h, and right after the treatment, they were assayed for osmotic avoidance behavior.n≥10; *P<0.05 (ANOVA); Error bars: s.e.m. (f) Reducing the level of endogenous H2O2in ASH neurons suppresses osmotic avoidance behavior. Transgenic expression of the catalase genectl-2in ASH neurons suppressed osmotic avoidance behavior. H2O2: 0.1 μM.n≥10; *P<0.05 (ANOVA); Error bars: s.e.m. Note: 0.1 μM H2O2was used to induce potentiation of osmotic avoidance behavior and ASH neuron sensory response throughout the paper unless otherwise indicated. Figure 1: Low doses of H 2 O 2 promote osmotic avoidance behavior. ( a ) Low doses of H 2 O 2 promote osmotic avoidance behavior while high concentrations of H 2 O 2 inhibit it. Worms were pre-incubated with varying concentrations of H 2 O 2 for 2 h. After a brief recovery on seeded NGM plates (up to 2 h), worms were tested for avoidance response to glycerol. To avoid a ceiling effect which would mask behavioral potentiation, a non-saturating concentration of glycerol (0.5 M) was used to challenge the worm. n ≥20; * P <0.05, ** P <0.005 (ANOVA with Dunnett’s test); Error bars: s.e.m. ( b ) Exposing worms to H 2 O 2 for one hour is sufficient to induce behavioral potentiation. Worms were pre-treated with 0.1 μM of H 2 O 2 for varying durations of time. n ≥20; * P <0.05, ** P <0.005, *** P <0.0005 ( t test); Error bars: s.e.m. ( c ) The antioxidants NAC and BHA block H 2 O 2 -induced behavioral potentiation. BHA (butylated hydroxyanisole, 25 μM) and NAC (N-acetyl-cysteine, 1 mM) were included during H 2 O 2 (0.1 μM ) treatment. n ≥10; *** P <0.0005 (ANOVA); Error bars: s.e.m. ( d ) Transgenic expression of the catalase gene ctl-2 in ASH neurons blocks H 2 O 2 -induced behavioral potentiation. H 2 O 2 : 0.1 μM. The sra-6 promoter was used to drive expression of ctl-2 in ASH neurons. n ≥10; ** P <0.005 (ANOVA); Error bars: s.e.m. ( e ) Reducing the level of endogenous H 2 O 2 suppresses osmotic avoidance behavior. Worms were treated with BHA or NAC for 2 h, and right after the treatment, they were assayed for osmotic avoidance behavior. n ≥10; * P <0.05 (ANOVA); Error bars: s.e.m. ( f ) Reducing the level of endogenous H 2 O 2 in ASH neurons suppresses osmotic avoidance behavior. Transgenic expression of the catalase gene ctl-2 in ASH neurons suppressed osmotic avoidance behavior. H 2 O 2 : 0.1 μM. n ≥10; * P <0.05 (ANOVA); Error bars: s.e.m. Note: 0.1 μM H 2 O 2 was used to induce potentiation of osmotic avoidance behavior and ASH neuron sensory response throughout the paper unless otherwise indicated. Full size image To verify whether the observed potentiation of behavioral responses was caused by H 2 O 2 , we tested the effect of N-acetyl-cysteine (NAC) and butylated hydroxyanisole (BHA), two commonly used antioxidants [13] . Both antioxidants blocked H 2 O 2 -induced behavioral potentiation ( Fig. 1c ). To provide further evidence, we took a genetic approach by overexpressing catalase in worms. Catalase specifically removes H 2 O 2 in the cell, antagonizing the action of H 2 O 2 (ref. 14 ). Overexpression of the C. elegans catalase gene ctl-2 as a transgene in ASH neurons, which mediate osmosensation [10] , [11] , abolished the ability of H 2 O 2 to induce behavioral potentiation ( Fig. 1d ). These results provide further evidence that H 2 O 2 treatment can potentiate osmotic avoidance behavior. Reducing endogenous H 2 O 2 level suppresses sensory behavior As H 2 O 2 treatment can potentiate osmotic avoidance behavior, we wondered if reducing the H 2 O 2 level suppresses this behavior. To test this, we treated worms with BHA and NAC, two commonly used H 2 O 2 scavengers. To better evaluate the effect of BHA and NAC, we modified the protocol by assaying the behavior right after the treatment (see Methods). We found that BHA and NAC treatment suppressed osmotic avoidance behavior ( Fig. 1e ), suggesting that endogenous H 2 O 2 may have a role in potentiating this sensory behavior. To interrogate the role of H 2 O 2 in ASH neurons, we assayed worms overexpressing ctl-2 as a transgene specifically in ASH neurons, as catalase specifically removes H 2 O 2 . We found that this transgene suppressed osmotic avoidance behavior ( Fig. 1f ). These results provide further evidence supporting a role of H 2 O 2 in promoting osmotic avoidance behavior. H 2 O 2 promotes sensory neuron function To investigate the neuronal mechanisms underlying H 2 O 2 -induced behavioral potentiation, we examined the function of ASH sensory neurons [10] , [11] . Calcium imaging experiments showed that H 2 O 2 treatment potentiated the response of ASH neurons to high osmolarity solution (glycerol) ( Fig. 2a,b ). This potentiation effect was abolished by the antioxidants NAC and BHA ( Fig. 2c–f ), as well as by a transgene overexpressing the catalase gene ctl-2 in ASH neurons ( Fig. 2g,h ). These data indicate that exposure to H 2 O 2 promoted ASH neuron function, providing a neuronal basis underlying H 2 O 2 -induced behavioral potentiation. 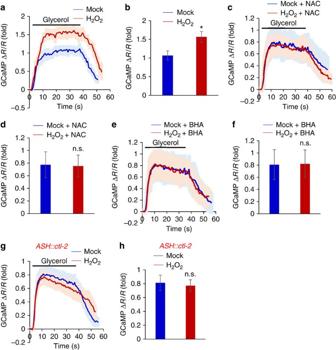Figure 2: H2O2treatment promotes ASH neuron function. (a,b) H2O2treatment potentiates the sensory response of ASH neurons. To enable ratiometric calcium imaging, GCaMP6 and mCherry were co-expressed in ASH neurons as a transgene using thesra-6promoter. Worms were pre-treated with H2O2(0.1 μM) for 2 h, and ASH neurons were recorded for their response to glycerol (0.5 M). Shades along the calcium traces in (a) represent error bars (s.e.m.). Bar graph in (b) summarizes the data in (a).n≥18; *P<0.05 (ANOVA); Error bars: s.e.m. (c–f) The antioxidants NAC and BHA block H2O2-induced potentiation of ASH sensory response. NAC or BHA was included during H2O2treatment. Calcium imaging of ASH neurons was performed as described in (a). Shades along the traces in (c) and (e) represent error bars (s.e.m.). Bar graph in (d) and (f) summarizes the data in (c) and (e), respectively.n≥8 (ANOVA); Error bars: s.e.m. (g,h) Transgenic expression of the catalase genectl-2blocks H2O2-induced potentiation of ASH sensory response. Thesra-6promoter was used to drive expression ofctl-2in ASH neurons. Calcium imaging of ASH neurons was performed as described in (a). Shades along the traces in (g) represent error bars (s.e.m.). Bar graph in (h) summarizes the data in (g).n≥9 (ANOVA); Error bars: s.e.m. Figure 2: H 2 O 2 treatment promotes ASH neuron function. ( a , b ) H 2 O 2 treatment potentiates the sensory response of ASH neurons. To enable ratiometric calcium imaging, GCaMP6 and mCherry were co-expressed in ASH neurons as a transgene using the sra-6 promoter. Worms were pre-treated with H 2 O 2 (0.1 μM) for 2 h, and ASH neurons were recorded for their response to glycerol (0.5 M). Shades along the calcium traces in ( a ) represent error bars (s.e.m.). Bar graph in ( b ) summarizes the data in ( a ). n ≥18; * P <0.05 (ANOVA); Error bars: s.e.m. ( c – f ) The antioxidants NAC and BHA block H 2 O 2 -induced potentiation of ASH sensory response. NAC or BHA was included during H 2 O 2 treatment. Calcium imaging of ASH neurons was performed as described in ( a ). Shades along the traces in ( c ) and ( e ) represent error bars (s.e.m.). Bar graph in ( d ) and ( f ) summarizes the data in ( c ) and ( e ), respectively. n ≥8 (ANOVA); Error bars: s.e.m. ( g , h ) Transgenic expression of the catalase gene ctl-2 blocks H 2 O 2 -induced potentiation of ASH sensory response. The sra-6 promoter was used to drive expression of ctl-2 in ASH neurons. Calcium imaging of ASH neurons was performed as described in ( a ). Shades along the traces in ( g ) represent error bars (s.e.m.). Bar graph in ( h ) summarizes the data in ( g ). n ≥9 (ANOVA); Error bars: s.e.m. Full size image We also examined other types of sensory behaviors such as chemotaxis. Similarly, exposing worms to low doses of H 2 O 2 potentiated their attractive behavioral responses to odors (that is diacetyl), indicating that H 2 O 2 treatment promoted olfactory behavior ( Supplementary Fig. 3a ). The sensory activity of AWA olfactory neurons, which detect diacetyl [15] , was also potentiated by H 2 O 2 treatment as shown by calcium imaging ( Supplementary Fig. 3b,c ). These results demonstrate that H 2 O 2 exposure can promote both avoidance and attractive behaviors. For simplicity, we decided to focus on osmotic avoidance behavior for further characterizations. p38/MAPK signaling mediates the potentiation effect of H 2 O 2 What are the molecular mechanisms underlying H 2 O 2 -induced potentiation of sensory behavior and neuronal function? H 2 O 2 is known to stimulate MAPK signaling [16] , [17] . The C. elegans genome encodes all three major classes of MAPKs: ERK, JNK and p38 (refs 18 , 19 ). We found that loss of the p38 gene pmk-1 abolished the ability of H 2 O 2 to induce behavioral potentiation, while the closely related pmk-3 was not required ( Fig. 3a ). In addition, mutations in ERK ( mpk-1 and mpk-2 ) and JNK ( jnk-1 ) did not have a notable effect ( Fig. 3b ). This points to a specific role for pmk-1 in mediating H 2 O 2 -induced behavioral potentiation, consistent with a reported role of pmk-1 in oxidative stress signaling [20] . Expression of pmk-1 complementary DNA (cDNA) as a transgene in ASH neurons was sufficient to rescue the phenotype ( Fig. 3a ), indicating that PMK-1 acts in ASH neurons. We also examined the activity of ASH by calcium imaging, and found that H 2 O 2 treatment can no longer promote ASH sensory activity in pmk-1 mutant worms ( Fig. 3c–e ), a defect that can be rescued by a transgene expressing pmk-1 cDNA in ASH neurons ( Fig. 3c–e ). Thus, the p38 ortholog PMK-1 is required for H 2 O 2 -induced potentiation of sensory behavior and ASH neuron function. 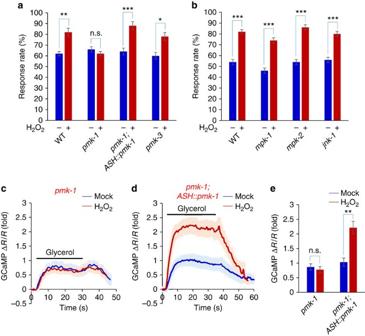Figure 3: H2O2-induced potentiation of sensory behavior and ASH neuron function requires the p38/MAPK PMK-1. (a) H2O2-induced behavioral potentiation requires PMK-1. Inpmk-1(km25)but notpmk-3(ok169)mutant worms, H2O2treatment failed to promote osmotic avoidance behavior. This defect was rescued by a transgene expressingpmk-1cDNA in ASH neurons driven by thesra-6promoter.n≥20; *P<0.05, **P<0.005, ***P<0.0005 (ANOVA); Error bars: s.e.m. (b) H2O2-induced behavioral potentiation does not require ERK (MPK-1 and MPK-2) or JNK (JNK-1).mpk-1(tm3476), mpk-2(tm3859)andjnk-1(gk7)mutant worms were tested.n≥10; ***P<0.0005 (ANOVA); Error bars: s.e.m. (c–e) H2O2-induced potentiation of ASH sensory response requires PMK-1. Inpmk-1mutant worms, H2O2treatment can no longer promote ASH calcium response to glycerol stimulus (c). This defect was rescued by a transgene expressingpmk-1cDNA in ASH neurons driven by thesra-6promoter (d). Shades along the traces in (c) and (d) represent error bars (s.e.m.). (e) summarizes the data in (c) and (d).n≥9; **P<0.005 (ANOVA); Error bars: s.e.m. Figure 3: H 2 O 2 -induced potentiation of sensory behavior and ASH neuron function requires the p38/MAPK PMK-1. ( a ) H 2 O 2 -induced behavioral potentiation requires PMK-1. In pmk-1(km25) but not pmk-3(ok169) mutant worms, H 2 O 2 treatment failed to promote osmotic avoidance behavior. This defect was rescued by a transgene expressing pmk-1 cDNA in ASH neurons driven by the sra-6 promoter. n ≥20; * P <0.05, ** P <0.005, *** P <0.0005 (ANOVA); Error bars: s.e.m. ( b ) H 2 O 2 -induced behavioral potentiation does not require ERK (MPK-1 and MPK-2) or JNK (JNK-1). mpk-1(tm3476), mpk-2(tm3859) and jnk-1(gk7) mutant worms were tested. n ≥10; *** P <0.0005 (ANOVA); Error bars: s.e.m. ( c – e ) H 2 O 2 -induced potentiation of ASH sensory response requires PMK-1. In pmk-1 mutant worms, H 2 O 2 treatment can no longer promote ASH calcium response to glycerol stimulus ( c ). This defect was rescued by a transgene expressing pmk-1 cDNA in ASH neurons driven by the sra-6 promoter ( d ). Shades along the traces in ( c ) and ( d ) represent error bars (s.e.m.). ( e ) summarizes the data in ( c ) and ( d ). n ≥9; ** P <0.005 (ANOVA); Error bars: s.e.m. Full size image p38 is activated by a conserved MAPK signaling cascade that has been extensively characterized biochemically and genetically in diverse organisms [17] , [18] , [19] , [21] . In C. elegans , the ASK1/MAPKKK ortholog NSY-1 and MKK/MAPKK ortholog SEK-1 are known to be in the cascade to activate p38/PMK-1 (refs 18 , 19 , 22 , 23 ). We thus tested NSY-1 and SEK-1. Loss of NSY-1 blocked the ability of H 2 O 2 to induce behavioral potentiation ( Fig. 4a ). RNAi of nsy-1 gene in ASH neurons using a transgene in wild-type background also blunted H 2 O 2 -induced behavioral potentiation ( Fig. 4a ). Apparently, NSY-1 is required in ASH neurons to mediate behavioral potentiation. Similarly, H 2 O 2 -induced behavioral potentiation was also absent in sek-1 mutant worms ( Fig. 4a ), and this phenotype can be rescued by a transgene expressing sek-1 cDNA in ASH neurons ( Fig. 4a ), demonstrating a requirement for SEK-1 in ASH neurons. Further evidence came from calcium imaging experiments. In nsy-1 mutant worms, H 2 O 2 treatment can no longer promote ASH sensory activity ( Fig. 4b,c ). RNAi of nsy-1 gene in ASH neurons using a transgene yielded a similar result ( Supplementary Fig. 4a,b ), suggesting that NSY-1 is required in ASH neurons to mediate neuronal potentiation. Similarly, we detected no potentiation of ASH sensory activity in sek-1 mutant worms ( Fig. 4d,e ), and this phenotype was rescued by a transgene expressing sek-1 cDNA in ASH neurons ( Supplementary Fig. 4c,d ). Thus, SEK-1 is also required for H 2 O 2 -induced potentiation of ASH sensory response. We conclude that the entire p38/MAPK signaling cascade is required for mediating H 2 O 2 -induced potentiation of sensory behavior and ASH neuron function. 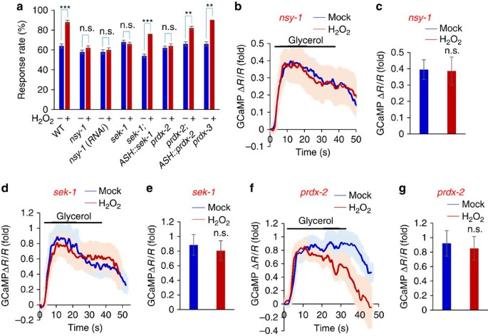Figure 4: H2O2-induced potentiation of sensory behavior and ASH neuron function requires peroxiredoxin-p38/PMK-1 signaling. (a) H2O2-induced behavioral potentiation requires NSY-1/ASK1, SEK-1/MKK, and PRDX-2/peroxiredoxin. Innsy-1(ok593), sek-1(km4)andprdx-2(gk169)mutant worms, H2O2treatment failed to promote osmotic avoidance behavior. RNAi ofnsy-1gene in ASH neurons of wild-type worms recapitulated the phenotype. This was done by expressingnsy-1RNAi as a transgene in ASH neurons under thesra-6promoter. Thesek-1andprdx-2mutant phenotype was rescued by a transgene expressingsek-1andprdx-2cDNA in ASH neurons driven by thesra-6promoter, respectively.n≥20; **P<0.005, ***P<0.0005 (ANOVA); Error bars: s.e.m. (b,c) H2O2-induced potentiation of ASH sensory response requires NSY-1. Innsy-1mutant worms, H2O2treatment can no longer promote ASH calcium response to glycerol stimulus (b). Shades along the traces in (b) represent error bars (s.e.m.). Bar graph in (c) summarizes the data in (b).n≥8; Error bars: s.e.m. (d,e) H2O2-induced potentiation of ASH sensory response requires SEK-1. Insek-1mutant worms, H2O2treatment can no longer promote ASH calcium response to glycerol stimulus (d). Shades along the traces in (d) represent error bars (s.e.m.). Bar graph in (e) summarizes the data in (d).n≥9; Error bars: s.e.m. (f,g) H2O2-induced potentiation of ASH sensory response requires PRDX-2. Inprdx-2mutant worms, H2O2treatment can no longer promote ASH calcium response to glycerol stimulus (f). Shades along the traces in (f) represent error bars (s.e.m.). Bar graph in (g) summarizes the data in (f).n≥8; Error bars: s.e.m. Figure 4: H 2 O 2 -induced potentiation of sensory behavior and ASH neuron function requires peroxiredoxin-p38/PMK-1 signaling. ( a ) H 2 O 2 -induced behavioral potentiation requires NSY-1/ASK1, SEK-1/MKK, and PRDX-2/peroxiredoxin. In nsy-1(ok593), sek-1(km4) and prdx-2(gk169) mutant worms, H 2 O 2 treatment failed to promote osmotic avoidance behavior. RNAi of nsy-1 gene in ASH neurons of wild-type worms recapitulated the phenotype. This was done by expressing nsy-1 RNAi as a transgene in ASH neurons under the sra-6 promoter. The sek-1 and prdx-2 mutant phenotype was rescued by a transgene expressing sek-1 and prdx-2 cDNA in ASH neurons driven by the sra-6 promoter, respectively. n ≥20; ** P <0.005, *** P <0.0005 (ANOVA); Error bars: s.e.m. ( b , c ) H 2 O 2 -induced potentiation of ASH sensory response requires NSY-1. In nsy-1 mutant worms, H 2 O 2 treatment can no longer promote ASH calcium response to glycerol stimulus ( b ). Shades along the traces in ( b ) represent error bars (s.e.m.). Bar graph in ( c ) summarizes the data in ( b ). n ≥8; Error bars: s.e.m. ( d , e ) H 2 O 2 -induced potentiation of ASH sensory response requires SEK-1. In sek-1 mutant worms, H 2 O 2 treatment can no longer promote ASH calcium response to glycerol stimulus ( d ). Shades along the traces in ( d ) represent error bars (s.e.m.). Bar graph in ( e ) summarizes the data in ( d ). n ≥9; Error bars: s.e.m. ( f , g ) H 2 O 2 -induced potentiation of ASH sensory response requires PRDX-2. In prdx-2 mutant worms, H 2 O 2 treatment can no longer promote ASH calcium response to glycerol stimulus ( f ). Shades along the traces in ( f ) represent error bars (s.e.m.). Bar graph in ( g ) summarizes the data in ( f ). n ≥8; Error bars: s.e.m. Full size image Role of peroxiredoxin in coupling H 2 O 2 to p38/MAPK signaling How is H 2 O 2 coupled to p38/MAPK signaling? Peroxiredoxin (PRDX) came to our attention, as recent studies have unveiled an increasingly important role for these ‘antioxidants’ in redox signaling [24] . In particular, 2-cys peroxiredoxin can serve as a ‘H 2 O 2 receptor’ [24] . In this case, H 2 O 2 oxidizes a specific Cys residue in peroxiredoxin, leading to the formation of a peroxiredoxin homodimer through disulfide bonds [24] , [25] . Dimerized peroxiredoxin can then activate ASK1/MAPKKK in the p38/MAPK pathway [25] , [26] . Thus, peroxiredoxin can potentially act as a H 2 O 2 sensor to functionally link H 2 O 2 to p38/MAPK signaling. The worm genome encodes two 2-cys peroxiredoxin genes: prdx-2 and prdx-3, and prdx-2 has been suggested as a H 2 O 2 sensor for lifespan regulation [25] . No defect was detected in prdx-3 mutant worms ( Fig. 4a ), indicating that prdx-3 is not required. By contrast, H 2 O 2 treatment failed to induce behavioral potentiation in prdx-2 mutant worms ( Fig. 4a ). Transgenic expression of prdx-2 cDNA in ASH neurons rescued the mutant phenotype ( Fig. 4a ). Thus, PRDX-2 acts in ASH neurons to mediate H 2 O 2 -induced behavioral potentiation. In addition, calcium imaging of ASH neurons in prdx-2 mutant worms failed to detect H 2 O 2 -induced potentiation of ASH sensory activity ( Fig. 4f,g ), and this defect can be rescued by a transgene expressing prdx-2 cDNA in ASH neurons ( Supplementary Fig. 4e,f ). These results identify PRDX-2/peroxiredoxin as a key molecule that couples H 2 O 2 to p38/MAPK signaling. AKT-1 acts downstream of p38/MAPK Having identified a key role for the peroxiredoxin-p38/MAPK signaling pathway, we then wondered which genes act downstream of this signaling pathway to mediate H 2 O 2 -induced potentiation of sensory behavior and ASH neuron function. In redox signaling, the transcription factor Nrf2 is well known to mediate oxidative stress signaling by turning on a host of antioxidant genes to combat oxidative insults [27] . Interestingly, p38/MAPK is known to activate Nrf2 through phosphorylation [27] , [28] . We thus examined the sole C. elegans Nrf2 ortholog SKN-1 (ref. 29 ). In skn-1 mutant worms, H 2 O 2 lost the ability to induce behavioral potentiation ( Supplementary Fig. 5a ), while mutant worms lacking DAF-16/FOXO, a transcription factor also involved in oxidative stress signaling, still exhibited H 2 O 2 -induced behavioral potentiation ( Supplementary Fig. 5f ). This supports a role for SKN-1 in the pathway. We also found that H 2 O 2 treatment up-regulated the expression of gst-4 and gcs-1 ( Supplementary Fig. 5g,h ), two well-characterized SKN-1 target genes [30] , suggesting that exposure to low doses of H 2 O 2 was sufficient to trigger oxidative stress responses in worms. Much to our surprise, recording of ASH neurons by calcium imaging detected robust H 2 O 2 -induced potentiation of ASH sensory response in skn-1 mutant worms ( Supplementary Fig. 5b–e ). Apparently, SKN-1 is not required for H 2 O 2 -induced potentiation of ASH neuron function. These results can be explained by a requirement of SKN-1 in those cells that act downstream of the sensory neuron ASH in the neural circuitry to drive osmotic avoidance behavior, for example, interneurons, motor neurons and/or muscles. The lack of a critical role for Nrf2/SKN-1 in ASH neurons poses a challenge to unravel the signaling events downstream of p38/PMK-1. Clearly, p38/PMK-1 substrates other than Nrf2/SKN-1 are involved. We reasoned that those proteins critical for ASH sensory activity could be potential targets of p38/PMK-1. The TRPV channel OSM-9 thus came to our attention because it is the primary sensory channel in ASH neurons [11] , [31] , [32] . However, no putative p38 phosphorylation site is predicted in OSM-9. On the other hand, five putative AKT phosphorylation sites are found in OSM-9 (see below). As it has been well established that p38/MAPK can activate AKT through a kinase complex [33] , we explored a potential involvement of AKT in mediating H 2 O 2 -induced behavioral potentiation. Two akt genes are encoded by the C. elegans genome: akt-1 and akt-2 . AKT-2 does not appear to be involved, as H 2 O 2 treatment can still induce behavioral potentiation in akt-2 mutant worms ( Fig. 5a ). By contrast, H 2 O 2 treatment failed to do so in akt-1 mutant animals ( Fig. 5a ). Transgenic expression of akt-1 cDNA in ASH neurons rescued the mutant phenotype ( Fig. 5a ), uncovering a key role for AKT-1 in mediating H 2 O 2 -induced behavioral potentiation. Calcium imaging of ASH neurons in akt-1 mutant worms also revealed a severe defect in H 2 O 2 -induced potentiation of ASH sensory response ( Fig. 5b–d ), and this phenotype can be rescued by a transgene expressing akt-1 cDNA in ASH neurons ( Supplementary Fig. 4g,h ). These data identify an important role for AKT-1 in the pathway. 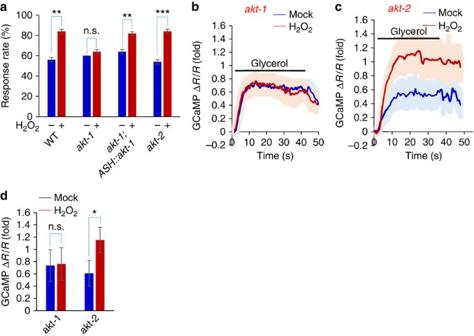Figure 5: H2O2-induced potentiation of sensory behavior and ASH neuron function requires AKT-1. (a) H2O2-induced behavioral potentiation requires AKT-1 but not AKT-2. Inakt-1(mg306)but notakt-2(ok391)mutant worms, H2O2treatment failed to promote osmotic avoidance behavior. This phenotype was rescued by a transgene expressingakt-1cDNA in ASH neurons driven by thesra-6promoter.n≥20; **P<0.005, ***P<0.0005 (ANOVA); Error bars: s.e.m. (b–d) H2O2-induced potentiation of ASH sensory response requires AKT-1 but not AKT-2. Inakt-1mutant worms, H2O2treatment can no longer promote ASH calcium response to glycerol stimulus (b). No such defect was detected inakt-2(k391)mutant worms. Shades along the traces in (b) and (c) represent error bars (s.e.m.). Bar graph in (d) summarizes the data in (b) and (c).n≥9; Error bars: s.e.m. *P<0.05 (ANOVA). Figure 5: H 2 O 2 -induced potentiation of sensory behavior and ASH neuron function requires AKT-1. ( a ) H 2 O 2 -induced behavioral potentiation requires AKT-1 but not AKT-2. In akt-1(mg306) but not akt-2(ok391) mutant worms, H 2 O 2 treatment failed to promote osmotic avoidance behavior. This phenotype was rescued by a transgene expressing akt-1 cDNA in ASH neurons driven by the sra-6 promoter. n ≥20; ** P <0.005, *** P <0.0005 (ANOVA); Error bars: s.e.m. ( b – d ) H 2 O 2 -induced potentiation of ASH sensory response requires AKT-1 but not AKT-2. In akt-1 mutant worms, H 2 O 2 treatment can no longer promote ASH calcium response to glycerol stimulus ( b ). No such defect was detected in akt-2(k391) mutant worms. Shades along the traces in ( b ) and ( c ) represent error bars (s.e.m.). Bar graph in ( d ) summarizes the data in ( b ) and ( c ). n ≥9; Error bars: s.e.m. * P <0.05 (ANOVA). Full size image Taken altogether, our data suggest that PDRX-2, MAPK pathway and AKT-1 form a signaling cascade to mediate the beneficial effect of H 2 O 2 . Though the upstream-downstream relationship between these molecules has been very well characterized biochemically in diverse organisms, we sought to gather some genetic evidence to further confirm such relationship through epistatic analysis. To do so, it is important to have both gain-of-function and loss-of-function mutant alleles. Two genes in this signaling cascade have both types of alleles available: nsy-1 /MAPKKK and akt-1 /AKT [34] , [35] . Worms carrying gain-of-function alleles of nsy-1 or akt-1 showed enhanced responses to high osmolarity solution ( Supplementary Fig. 6a ), consistent with a role for these two genes in promoting osmotic avoidance behavior. As reducing the level of endogenous H 2 O 2 by a transgene overexpressing the catalase CTL-2 inhibited osmotic avoidance behavior ( Fig. 1f and Supplementary Fig. 6a ), we tested whether nsy-1 and akt-1 gain-of-function alleles can suppress this inhibitory effect, and found that they did ( Supplementary Fig. 6a ). This is consistent with the view that MAPK pathway and AKT act downstream of H 2 O 2 . We also found that akt-1 loss-of-function mutation suppressed the phenotype of nsy-1 gain-of-function mutant worms ( Supplementary Fig. 6b ), and vice versa ( Supplementary Fig. 6c ), consistent with the notion that AKT acts downstream of MAPK pathway. These epistatic analyses lend support to our model. The detrimental effect of H 2 O 2 does not require PMK-1 or AKT-1 As treating worms with high concentrations of H 2 O 2 (for example 1 mM) suppressed osmotic avoidance behavior ( Fig. 1a ), we wondered if this detrimental effect of H 2 O 2 is also mediated by the same signaling cascade. Interestingly, while H 2 O 2 -induced suppression of osmotic avoidance behavior still required the ‘H 2 O 2 receptor’ PRDX-2, it did not depend on MAPK/PMK-1 ( Supplementary Fig. 7a ); nor did it rely on AKT-1 ( Supplementary Fig. 7a ). Calcium imaging of ASH neurons yielded similar results ( Supplementary Fig. 7b–i ). We thus suggest that the beneficial and detrimental effects of H 2 O 2 are likely to be mediated by different signaling pathways. A key role of the putative AKT site Thr10 in OSM-9 As OSM-9 is predicted to possess five putative AKT phosphorylation sites and it is also the primary sensory channel in ASH neurons, we hypothesize that OSM-9 may be a downstream target of AKT. To test this idea, we asked whether any of those putative AKT phosphorylation sites in OSM-9 is critical for H 2 O 2 -induced behavioral potentiation ( Fig. 6a ). Among the five putative AKT sites, one is located at the N-terminal end of OSM-9 while the other four are found at the C-terminus ( Fig. 6a ). We mutated all four C-terminal AKT sites in osm-9 cDNA from S/T to A, and introduced this ‘quad mutant’ as a transgene in ASH neurons in the osm-9 mutant background. As reported previously [11] , [31] , osm-9 mutant worms did not respond to high osmolarity stimulus ( Fig. 6b ) (note: the basal response rate in the mutant arose from stimulus-independent spontaneous reversal events). As was the case with osm-9 wild-type transgene, osm-9(quad mutant) transgene expressed in ASH neurons can rescue osmotic avoidance behavioral response in naive worms, as well as behavioral potentiation in H 2 O 2 -treated worms ( Fig. 6b ). We conclude that the four putative AKT sites at the C-terminal end of OSM-9 are not required for H 2 O 2 -induced behavioral potentiation. 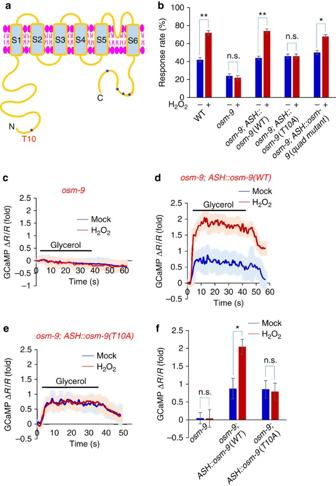Figure 6: The putative AKT phosphorylation site T10 in OSM-9 is required for H2O2-induced potentiation of sensory behavior and ASH function. (a) Schematic of OSM-9 domain organization. Both the N and C-terminal fragments of OSM-9 are located intracellularly. Asterisks denote the putative AKT phosphorylation sites, with one at the N-terminus (T10) and the other four at the C-terminus (T769, T771, T787 and S839). These sites are predicted by Scansite. The N-terminal point mutation T10A is indicated. (b) The putative AKT phosphorylation site T10 in OSM-9 is required for H2O2-induced behavioral potentiation.osm-9(ky10)mutants failed to respond to glycerol stimulus. The basal response rate in the mutant arose from spontaneous reversal events that are present in the absence of glycerol stimulation. Wild-type and mutant forms of OSM-9 were expressed as transgenes in ASH neurons under thesra-6promoter. Wild-typeosm-9transgene (ASH::osm-9), as well asosm-9transgene with all the four putative C-terminal AKT sites mutated (that isASH::osm-9(quad mutant)) rescued both the basal and H2O2-induced potentiation of osmotic avoidance response. However,osm-9transgene harboring the point mutation T10A (that isASH::osm-9(T10A)) failed to rescue H2O2-induced potentiation of osmotic avoidance response, though it rescued the basal avoidance behavior.n≥10; *P<0.05, **P<0.005 (ANOVA); Error bars: s.e.m. (c–f) The putative AKT phosphorylation site T10 in OSM-9 is required for H2O2-induced potentiation of ASH sensory response. Inosm-9mutant worms, ASH neurons did not respond to glycerol (c), and this defect was rescued by wild-typeosm-9transgene (d). Wild-typeosm-9transgene also rescued H2O2-induced potentiation of ASH sensory response (d). However,osm-9transgene with the point mutation T10A (that isASH::osm-9(T10A)) did not rescue H2O2-induced potentiation of ASH sensory response, though it rescued the basal glycerol sensory response in ASH neurons(e). Shades along the traces in (c–e) represent error bars (s.e.m.). Bar graph in (f) summarizes the data in (c–e).n≥8; Error bars: s.e.m. *P<0.05 (ANOVA). Figure 6: The putative AKT phosphorylation site T10 in OSM-9 is required for H 2 O 2 -induced potentiation of sensory behavior and ASH function. ( a ) Schematic of OSM-9 domain organization. Both the N and C-terminal fragments of OSM-9 are located intracellularly. Asterisks denote the putative AKT phosphorylation sites, with one at the N-terminus (T10) and the other four at the C-terminus (T769, T771, T787 and S839). These sites are predicted by Scansite. The N-terminal point mutation T10A is indicated. ( b ) The putative AKT phosphorylation site T10 in OSM-9 is required for H 2 O 2 -induced behavioral potentiation. osm-9(ky10) mutants failed to respond to glycerol stimulus. The basal response rate in the mutant arose from spontaneous reversal events that are present in the absence of glycerol stimulation. Wild-type and mutant forms of OSM-9 were expressed as transgenes in ASH neurons under the sra-6 promoter. Wild-type osm-9 transgene ( ASH::osm-9 ), as well as osm-9 transgene with all the four putative C-terminal AKT sites mutated (that is ASH::osm-9(quad mutant) ) rescued both the basal and H 2 O 2 -induced potentiation of osmotic avoidance response. However, osm-9 transgene harboring the point mutation T10A (that is ASH::osm-9(T10A) ) failed to rescue H 2 O 2 -induced potentiation of osmotic avoidance response, though it rescued the basal avoidance behavior. n ≥10; * P <0.05, ** P <0.005 (ANOVA); Error bars: s.e.m. ( c – f ) The putative AKT phosphorylation site T10 in OSM-9 is required for H 2 O 2 -induced potentiation of ASH sensory response. In osm-9 mutant worms, ASH neurons did not respond to glycerol ( c ), and this defect was rescued by wild-type osm-9 transgene ( d ). Wild-type osm-9 transgene also rescued H 2 O 2 -induced potentiation of ASH sensory response ( d ). However, osm-9 transgene with the point mutation T10A (that is ASH::osm-9(T10A) ) did not rescue H 2 O 2 -induced potentiation of ASH sensory response, though it rescued the basal glycerol sensory response in ASH neurons( e ). Shades along the traces in ( c – e ) represent error bars (s.e.m.). Bar graph in ( f ) summarizes the data in ( c – e ). n ≥8; Error bars: s.e.m. * P <0.05 (ANOVA). Full size image We then turned our attention to the putative AKT site at the N-terminus of OSM-9. We generated a transgene osm-9 ( T10A ) harboring a point mutation with this site changed to A ( Fig. 6a ). As was the case with wild-type osm-9 transgene, expression of osm-9 ( T10A ) transgene in ASH neurons of osm-9 mutant worms rescued the basal osmotic behavioral response ( Fig. 6b ). This shows that the basic function of OSM-9 was not compromised by T10A mutation. However, this osm-9 ( T10A ) transgene failed to rescue H 2 O 2 -induced behavioral potentiation ( Fig. 6b ), revealing a requirement for the putative phosphorylation site T10 in mediating H 2 O 2 -induced behavioral potentiation. To gather functional evidence, we conducted calcium imaging experiments. Similar to wild-type osm-9 transgene ( Fig. 6c,d ), osm-9 ( T10A ) transgene also rescued the basal ASH sensory response in osm-9 mutant worms ( Fig. 6e,f ), supporting the notion that the basic function of OSM-9 was not compromised by T10A mutation. However, this osm-9 ( T10A ) transgene failed to rescue H 2 O 2 -induced potentiation of ASH sensory response ( Fig. 6e,f ). By contrast, osm-9(quad mutant) transgene, in which all four C-terminal AKT sites were mutated, rescued H 2 O 2 -induced potentiation of ASH sensory response ( Supplementary Fig. 8 ). This set of experiments uncovers a specific role for the putative AKT phosphorylation site T10 in OSM-9 in mediating H 2 O 2 -induced potentiation of sensory behavior and ASH neuron function. To provide additional evidence, we recorded OSM-9-mediated sensory current by patch-clamp. Perfusion of glycerol-containing high osmolarity solution evoked an inward current in ASH neurons ( Supplementary Fig. 9a,b ). H 2 O 2 treatment potentiated this current ( Supplementary Fig. 9a,b ), which is consistent with our behavioral and calcium imaging data. Using the same strategy as behavioral analysis and calcium imaging, we introduced transgenes expressing osm-9 cDNA in ASH neurons in osm-9 mutant background. Wild-type osm-9 transgene retained the ability to mediate H 2 O 2 -induced potentiation of sensory current ( Supplementary Fig. 9c,d ). By contrast, the osm-9(T10A) transgene, which encompasses a point mutation disrupting the putative AKT phosphorylation site, lost the ability to mediate H 2 O 2 -induced potentiation of sensory current ( Supplementary Fig. 9e,f ). This patch-clamp data presents additional evidence supporting a key role for the putative AKT site T10 in OSM-9 in mediating H 2 O 2 -induced potentiation of ASH sensory response. AKT-1 phosphorylates OSM-9 at Thr10 in vitro The above data raised the intriguing possibility that the TRPV channel OSM-9 may be a substrate for AKT-1 kinase. To test this model, we performed an in vitro kinase assay. We produced the N-terminal fragment of OSM-9 as a GST fusion protein (that is GST-N-OSM-9) and purified it from bacteria lysate ( Fig. 7a ). The pan-kinase substrate MBP served as a positive control ( Fig. 7a,b ). Notably, AKT-1 transfected in HEK293 cells can phosphorylate GST-N-OSM-9 but not GST alone or GST-N-OSM-9(T10A) that harbors the point mutation T10A ( Fig. 7b ). Thus, AKT-1 can phosphorylate OSM-9 in vitro , identifying OSM-9 as a substrate for AKT-1. 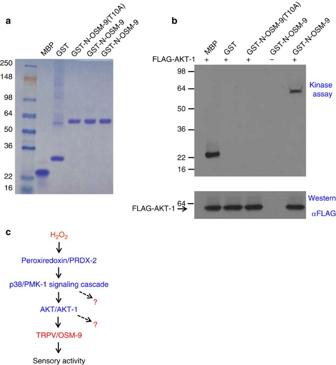Figure 7: AKT-1 phosphorylates OSM-9in vitro. (a)In vitroproduction of GST fusion proteins of OSM-9. The N-terminal fragment of wild-type and point mutant (T10A) of OSM-9 was fused to GST, expressed and purified from bacterial strain BL21. Shown is a SDS-PAGE gel stained by Coomassie blue. The pan-kinase substrate MBP and GST alone were also shown. (b) AKT-1 phosphorylates OSM-9 in anin vitrokinase assay. FLAG-tagged AKT-1 was transfected in HEK293T cells. After pull-down by anti-FLAG affinity beads, AKT-1 was tested for its ability to phosphorylate purified MBP, GST, and GST fusion proteins using (γ-32P)ATP as the substrate. Top panel: autoradiograph. Bottom panel: Western blot showing the amount of AKT-1 used in each experiment. (c) A schematic model illustrating the signaling pathway that mediates H2O2-induced potentiation of neuronal activity. Question marks indicate that additional substrates may exist. Figure 7: AKT-1 phosphorylates OSM-9 in vitro . ( a ) In vitro production of GST fusion proteins of OSM-9. The N-terminal fragment of wild-type and point mutant (T10A) of OSM-9 was fused to GST, expressed and purified from bacterial strain BL21. Shown is a SDS-PAGE gel stained by Coomassie blue. The pan-kinase substrate MBP and GST alone were also shown. ( b ) AKT-1 phosphorylates OSM-9 in an in vitro kinase assay. FLAG-tagged AKT-1 was transfected in HEK293T cells. After pull-down by anti-FLAG affinity beads, AKT-1 was tested for its ability to phosphorylate purified MBP, GST, and GST fusion proteins using (γ- 32 P)ATP as the substrate. Top panel: autoradiograph. Bottom panel: Western blot showing the amount of AKT-1 used in each experiment. ( c ) A schematic model illustrating the signaling pathway that mediates H 2 O 2 -induced potentiation of neuronal activity. Question marks indicate that additional substrates may exist. Full size image Owing to their deleterious effects on cellular functions, ROS have been implicated in a large variety of human diseases particularly neurodegenerative diseases [2] , [4] . In the current study, we demonstrate that unlike the commonly observed adverse effects of ROS, low doses of H 2 O 2 can in fact promote sensory behavior and potentiate sensory neuron function in C. elegans , revealing a beneficial role of ROS in the nervous system. We also show that reducing the level of endogenous H 2 O 2 compromises sensory behavior, suggesting that the role of H 2 O 2 in promoting neuronal function is physiological. Such an effect of ROS may benefit the survival of C. elegans . For example, ROS are often associated with harsh environments. Sensitization of sensory neurons, such as the polymodal neuron ASH, by ROS would render the animals more responsive to noxious cues and thereby facilitate their escape from harsh environments. Meanwhile, as ROS can also promote the activity of chemosensory neurons such as AWA that detects food sources, this effect may also help the animals to approach pleasant environments. Our results point to a model in which H 2 O 2 promotes sensory behavior and ASH neuron function through a peroxiredoxin-p38/MAPK signaling axis ( Fig. 7c ). In this model, we propose that peroxiredoxin acts as a H 2 O 2 sensor that transduces information through p38/MAPK signaling which in turn signals to AKT and the sensory channel OSM-9/TRPV in ASH neurons ( Fig. 7c ), and that AKT regulates the OSM-9/TRPV sensory channel by phosphorylating its N-terminus. As all the members in the peroxiredoxin-p38/MAPK signaling pathway are evolutionarily conserved across phylogeny, our results raise the intriguing possibility that H 2 O 2 may play a similar role in regulating brain function in other organisms. In addition to their role in the brain, ROS have been proposed to underlie cellular senescence of other cell types and affect organismal aging [36] . Interestingly, recent studies in C. elegans show that accumulation of ROS is not causal in the aging process and a mild increase in ROS production in mitochondria of ASI diet-sensitive neurons may even prolong lifespan through mitohormesis [6] , [7] , [36] , [37] . Though the underlying mechanisms are not well understood, p38/PMK-1 and SKN-1/Nrf2 are found to be involved [20] , [37] , [38] . This reveals a common role of p38/PMK-1 in mediating both ROS-mediated extension of lifespan and potentiation of neuronal function. Nevertheless, the signaling events downstream of p38/PMK-1 appear to be different in these two processes. High doses of H 2 O 2 compromise sensory behavior and sensory neuron function. One possibility is that this deleterious effect of H 2 O 2 may result from its non-specific modification of proteins, nucleic acids and lipids. Interestingly, we find that this effect can also be blocked by loss of PRDX-2, indicating that it involves specific genes. On the other hand, mutations in p38/PMK-1 and AKT-1 cannot block this detrimental effect. Thus, other signaling pathways are probably also involved. We suggest that under low concentrations, ROS may primarily function as signaling molecules regulating specific cellular pathways, the outcome of which could be beneficial, while under high doses, ROS would become harmful by acting as signaling molecules and also by non-specifically modifying proteins, lipids and nucleic acids. We identify the TRPV channel OSM-9 as a critical substrate for the peroxidoxin-p38/MAPK signaling pathway in ASH sensory neurons. Some TRP channels such as TRPA, TRPV and TRPC channels can be directly regulated by ROS through oxidation [39] . We thus do not rule out the possibility that OSM-9 may also be regulated by this mechanism. It should be noted that OSM-9 is probably not the only target of the peroxidoxin-p38/MAPK signaling pathway in ASH neurons. In other words, this signaling cascade may impinge on additional substrates in ASH, but the identities of which remain to be identified ( Fig. 7c ). These additional substrates may contribute to H 2 O 2 -induced potentiation of sensory behavior and ASH neuron function. It is also possible that peroxiredoxin-p38/MAPK signaling may recruit different sets of substrates in different classes of neurons. Lastly, we do not rule out the possibility that pathways other than peroxiredoxin-p38/MAPK may contribute to the observed beneficial effect of H 2 O 2 . Future effort is needed to address these intriguing questions. The current study unveils unexpected complexity of the action of ROS in the nervous system, providing an entry point to understanding the multifaceted roles of ROS in health and disease. Strains See Supplementary Table 1 . Behavioral assays Osmotic avoidance behavior was carried out at 20 °C using a drop test assay as described previously [40] , [41] . Day 1 adult hermaphrodites were tested. We placed a small drop of glycerol-containing solution (M9) in the path of a worm moving forward. A positive response was scored if the worm stopped forward movement and also initiated a reversal that lasted at least half a head swing. The assay was conducted on NGM plates without bacteria. To avoid a ceiling effect that would mask behavioral potentiation, we used a non-saturating concentration of glycerol (for example 0.25–0.5 M) unless otherwise specified. Each worm was tested five times and a response rate was calculated for each animal. In general, 10–20 worms were assayed for each experiment ( n number=10–20 worms), which should be sufficient based on power analysis. Chemotaxis assay was performed using the standard protocol described previously [15] . To avoid a ceiling effect, we used a non-saturating concentration of diacetyl (50,000 dilution) unless otherwise indicated. To treat worms with H 2 O 2 , we incubated them with varying concentrations of H 2 O 2 diluted in M9 buffer for 2 h. Fresh OP50 bacteria were included in M9 buffer to prevent starvation during H 2 O 2 treatment. After treatment, worms were allowed to recover on seeded NGM plates for up to 2 h before behavioral, imaging and patch-clamp analysis. Mock-treated worms were used as a control. We also tested untreated worms (left on seeded NGM plates for 2 h) and found no difference from mock-treated worms ( Supplementary Fig. 1 ). To test whether reducing the level of endogenous H 2 O 2 would affect osmotic avoidance behavior, we treated worms with BHA or NAC for 2 h (OP50 included) and then assayed worms right after the treatment, since recovering worms on NGM plates would allow BHA and NAC to diffuse out, which would presumably lead to a rebound in H 2 O 2 level inside the cell. 0.1 μM H 2 O 2 was used to induce potentiation of osmotic avoidance behavior and ASH neuron sensory response throughout the paper unless otherwise indicated. Calcium imaging A microfluidic system was used to perform calcium imaging on Day 1 adult worms [42] . Worms were loaded onto a microfluidic chip mounted on an upright microscope (Olympus BX51WI), and incubated in standard bath solution (in mM): 145 NaCl, 2.5 KCl, 1 CaCl 2 , 1 MgCl 2 , 20 glucose and 5 HEPES (320 mOsm; pH adjusted to 7.3). The images were acquired with a Roper Coolsnap CCD camera and analysed with MetaFluor software (Molecular Devices, Inc.). GCaMP6 and DsRed were co-expressed as a transgene in ASH under the sra-6 promoter to enable ratiometric imaging using blue and red light [43] , [44] , [45] . As ASH neurons are photosensitive [46] , we first exposed them to blue light for 2 min to bleach their intrinsic photosensitivity before applying chemical stimuli. The peak fold change in the ratio of G-CaMP/DsRed fluorescence was analysed. Each worm was only imaged once. Electrophysiology Whole-cell recordings were performed on an upright microscope (BX51WI) with an EPC-10 amplifier [45] , [47] , [48] . Worms were glued and dissected on a sylgard-coated coverglass to expose ASH neurons. Bath solution (in mM): 145 NaCl, 2.5 KCl, 1 CaCl 2 , 1 MgCl 2 , 20 glucose and 5 HEPES (320 mOsm; pH adjusted to 7.3). Pipette solution: 115 K-gluconate, 15 KCl, 1 MgCl 2 , 10 HEPES, 0.25 CaCl 2 , 20 sucrose, 5 BAPTA, 5 Na 2 ATP and 0.5 NaGTP (315 mOsm; pH adjusted to 7.2). DsRed and YFP fluorescence markers were expressed as a transgene ( xuEx631 ) to label and identify ASH neurons for recording. Clamping voltage: −60 mV. Series resistance and membrane capacitance were both compensated during recording. Biochemistry GST fusion proteins were expressed and purified from BL21 bacteria using the standard protocol [49] . Briefly, after IPTG induction (1 mM, 5 h), bacteria were pelleted and resuspended in TEN buffer (10 mM Tris, pH 8.0, 1 mM EDTA, 0.4% NP-40 and 1 mM DTT), and lysed by sonication. GST fusions were then purified using glutathione beads. To prepare for kinase assay, worm FLAG AKT-1 was cloned into pcDNA3 vector and transfected into HEK293T cells. Cells were lysed with lysis buffer (100 mM Tris pH 7.5, 1% NP-40, 10% glycerol, 130 mM sodium chloride, 5 mM MgCl 2 , 1 mM sodium vanadate, 1 mM NaF and 1 mM EDTA) supplemented with protease inhibitor cocktail (Roche). FLAG-AKT-1 was then pulled down by immunoprecipitation with anti-FLAG affinity beads. In vitro kinase assay was performed by incubating GST fusion proteins and FLAG-AKT-1-bound affinity beads in 50 μl kinase buffer (50 mM MOPS pH 7.2, 50 mM NaCl, 25 mM b-glycerolphosphate, 10 mM MgCl 2 , 1 mM sodium vanadate, 1 mM NaCl and 100 uM ATP). 5 μCi of (γ 32 P)ATP and lipid activator mix (Millipore) were included in the kinase reaction. The reaction was stopped by adding 5 × SDS–polyacrylamide gel electrophoresis (SDS–PAGE) sample buffer, and the proteins were separated by SDS–PAGE and transferred to nitrocellulose membrane followed by autoradiography and Western probed with an anti-FLAG antibody (1:5,000 dilution, Cat#. F4042, Sigma). The Western image in Supplementary Fig. 7b was cropped for presentation, and the full size image is presented in Supplementary Fig. 10 . Data Availability All custom strains have been made available at http://cbs.umn.edu/cgc/home or http://shigen.nig.ac.jp/c.elegans/ . Additional modified strains can be accessed upon request. The data that support the findings of this study are available from the corresponding author on reasonable request. How to cite this article : Li, G. et al . Promotion of behavior and neuronal function by reactive oxygen species in C. elegans . Nat. Commun. 7 , 13234 doi: 10.1038/ncomms13234 (2016). Publisher's note: Springer Nature remains neutral with regard to jurisdictional claims in published maps and institutional affiliations.